Poly(ADP-ribose) controls DE-cadherin-dependent stem cell maintenance and oocyte localization Within the short span of the cell cycle, poly(ADP-ribose) (pADPr) can be rapidly produced by poly(ADP-ribose) polymerases and degraded by poly(ADP-ribose) glycohydrolases. Here we show that changes in association between pADPr and heterogeneous nuclear ribonucleoproteins (hnRNPs) regulate germline stem cell (GSC) maintenance and egg chamber polarity during oogenesis in Drosophila . The association of pADPr and Hrp38, an orthologue of human hnRNPA1, disrupts the interaction of Hrp38 with the 5′-untranslated region of DE-cadherin messenger RNA, thereby diminishing DE-cadherin translation in progenitor cells. Following the reduction of DE-cadherin level, GSCs leave the stem cell niche and differentiate. Defects in either pADPr catabolism or Hrp38 function cause a decrease in DE-cadherin translation, leading to a loss of GSCs and mislocalization of oocytes in the ovary. Taken together, our findings suggest that Hrp38 and its association with pADPr control GSC self-renewal and oocyte localization by regulating DE-cadherin translation. In Drosophila , oogenesis begins with the asymmetrical division of one germline stem cell (GSC) into two: one GSC for self-renewal and one cystoblast that differentiates within the germarium [1] . Maintenance of GSCs is controlled by several pathways [2] , [3] , [4] , [5] , [6] , including the regulation of DE-cadherin expression that promotes anchoring of GSC to its niche through adherens junctions (AJs) [6] . Subsequently, one GSC daughter cell, the cystoblast, loses contact with the GSC niche and divides four times to form a cyst consisting of 15 nurse cells and an oocyte [7] . On completion of proliferation, migration and differentiation of follicle stem cells in the middle of the germarium, a monolayer of follicle cells surrounds this 16-cell cyst to form an egg chamber [8] . During the last germarial stage, the elevated DE-cadherin-dependent adhesion between the oocyte and its surrounding follicle cells helps anchor the oocyte in the posterior pole, establishing the anterior–posterior axis of an egg chamber [9] , [10] . Heterogeneous nuclear ribonucleoproteins (HnRNPs) are ubiquitous RNA-binding proteins associated with pre-messenger RNA(mRNA)/mRNA in the nucleus and/or cytoplasm of the cell during transcription and post-transcriptional possesses [11] , [12] , [13] , [14] , [15] , [16] , [17] . Poly(ADP-ribose) (pADPr), a polymer formed from 2 to 200 ADP-ribose units, is produced by poly(ADP-ribose) polymerase-1 (PARP1) using NAD as a substrate [19] . Non-covalent association of PARP1–pADPr with hnRNP decorates this protein with negative charges and prevents its binding to RNA [19] . This regulation depends on the activity of PARP1, which adds pADPr to proteins [19] , and poly(ADP-ribose) glycohydrolase (PARG), which removes pADPr [20] . Our present study demonstrates that pADPr association with hnRNPs controls DE-cadherin expression. We show that a high level of pADPr titrates Hrp38—an orthologue of human hnRNPA1—away from DE-cadherin mRNA and blocks Hrp38-dependent translation. Furthermore, we show that pADPr binding to Hrp38 is essential for GSC function and oocyte positioning during oogenesis. pADPr is enriched in Drosophila ovary We determined the level of pADPr accumulation in different tissues of adult Drosophila by western blotting. The largest amount of pADPr accumulated in the ovary, for which multiple bands of pADPr were observed ( Fig. 1a ). To track in vivo pADPr accumulation in the ovary, we cultured a dissected Drosophila ovary in the presence of biotinylated NAD ( b NAD). Previously, we reported that PARP1 converts b NAD into b pADPr [21] . We examined 437 germaria and observed 31 dividing GSCs, all exhibiting the highest level of biotin labelling ( Fig. 1b–d ). GSCs in the interphase did not incorporate any b NAD ( Fig. 1c,d ). Severe 'punctate' labelling by b NAD was detected in cystoblasts ( Fig. 1c,d , arrows). High levels of biotin labelling persisted during maturation of germline cysts starting from region 1 of germarium ( Fig. 1c–e ), yet labelling was depleted in the oocyte in stage 9 ( Fig. 1f ). These findings indicate the potential importance of pADPr turnover for progression of early oogenesis. 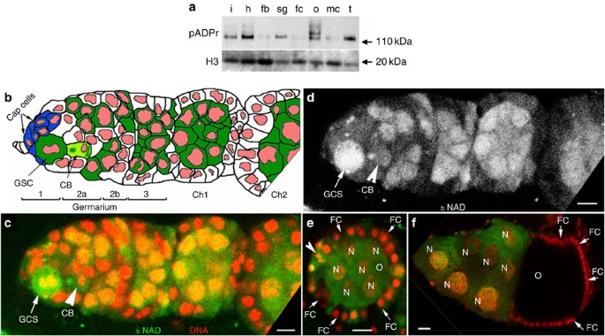Figure 1: pADPr accumulates in mitotic germline stem cell and cystoblast. (a) The comparison of total cellular pADPr level in different tissues ofDrosophilaadult by western blotting. The total protein from different tissues was immunoblotted with anti-pADPr antibody. The same blot was stripped and detected with anti-H3 antibody for loading control. fb: fat bodies; fc: female carcasses; h: heads; i: intestines; mc: male carcasses; o: ovaries; sg: salivary glands; t: testes. (b) Schematic illustration of anterior part ofDrosophilaovariole (matchingcandd). Cap cells (blue) form germline stem cell (GSC) niche. CB: cystoblast; Ch1,Ch2: egg chambers 1 and 2. Germline cells are shown in green. Nuclei are shown in red. (c–f) Incorporation of the biotinylated NAD (bNAD) intoin vitroculturedDrosophilaovary.bNAD was detected using Avidin-Rhodamine staining (green). DNA was detected using oligreen dye (red). Strong accumulation ofbNAD within dividing germline stem cell (GSC; arrow), cystoblast (CB; arrow) and in maturating germline cysts. (c) Germarium and egg chamber 1. (d) Germarium and egg chamber 1 (onlybNAD is shown). (e,f) Egg chamber stages 4 (e) and 9 (f). FC: follicle cells; N: nurse cells; O: oocyte. Arrowhead indicates follicle cell in mitosis. Scale bars, 10 μm. Figure 1: pADPr accumulates in mitotic germline stem cell and cystoblast. ( a ) The comparison of total cellular pADPr level in different tissues of Drosophila adult by western blotting. The total protein from different tissues was immunoblotted with anti-pADPr antibody. The same blot was stripped and detected with anti-H3 antibody for loading control. fb: fat bodies; fc: female carcasses; h: heads; i: intestines; mc: male carcasses; o: ovaries; sg: salivary glands; t: testes. ( b ) Schematic illustration of anterior part of Drosophila ovariole (matching c and d ). Cap cells (blue) form germline stem cell (GSC) niche. CB: cystoblast; Ch1,Ch2: egg chambers 1 and 2. Germline cells are shown in green. Nuclei are shown in red. ( c – f ) Incorporation of the biotinylated NAD ( b NAD) into in vitro cultured Drosophila ovary. b NAD was detected using Avidin-Rhodamine staining (green). DNA was detected using oligreen dye (red). Strong accumulation of b NAD within dividing germline stem cell (GSC; arrow), cystoblast (CB; arrow) and in maturating germline cysts. ( c ) Germarium and egg chamber 1. ( d ) Germarium and egg chamber 1 (only b NAD is shown). ( e , f ) Egg chamber stages 4 ( e ) and 9 ( f ). FC: follicle cells; N: nurse cells; O: oocyte. Arrowhead indicates follicle cell in mitosis. Scale bars, 10 μm. Full size image The Parg gene is required for oocyte localization As PARG removes pADPr to promote dynamic turnover of pADPr, we expected to find that PARG is required for normal oogenesis. Indeed, we detected Parg mRNAs in follicle and germline cells in wild-type ovaries using RNA in situ hybridization with an antisense Parg RNA probe ( Fig. 2a,b , Supplementary Methods ). Ectopically expressed PARG-EGFP (Enhanced GFP) was localized to the nucleoplasm of nurse cells and the oocyte in stage 7 egg chambers, confirming that PARG recycles pADPr in nuclei of the ovary cells ( Fig. 2c ). To test whether the Parg gene is essential for oogenesis, we generated Parg mutant clones in the ovary using the FRT/FLP system. Wild-type clones ( Fig. 2d ) as well as egg chambers with Parg mutant germline clones only ( n =73) or follicle cell clones only ( n =91) did not show oocyte mislocalization ( Fig. 2e,f ). However, egg chambers bearing Parg mutant clones, both in the follicle cells, including the polar cells, and the germline cells, exhibited mislocalization of the oocyte to its midpoint (36% ( n =45), Fig. 2g,h ). These results show that loss of Parg in both germline and polar cell clones is a precondition for oocyte mislocalization in the Parg mutant. 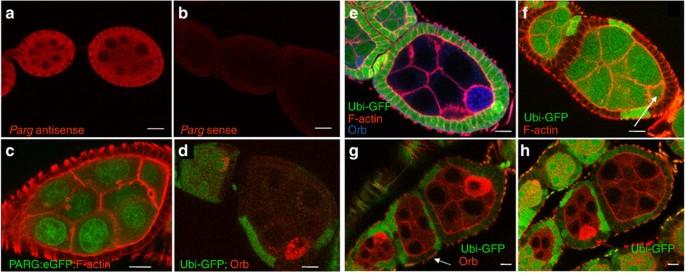Figure 2:Pargexpression in the ovary and mislocalization of the oocyte caused byPargmutant clones. The anterior pole of all egg chambers is to the left, and the posterior pole is to the right. (a)PargmRNA expression in the ovary of the wild type (y,w) detected by RNAin situhybridization usingPargantisense probe. (b) The control of RNAin situhybridization usingPargsense probe. (c) The expression of PARG-EGFP in the ovary induced by germline-specific GAL4 drivers. (d) The mock wild-type clones, including germline and polar follicle cells, showing the normal localization of the oocyte in the posterior. The oocyte is labelled with anti-orb antibody (red). The clones are generated from the female adults (FRT101/FRT101, ubi-GFP; FLP38/+) after heat shock. (e)Pargmutant germline clones showing the normal localization of the oocyte in the posterior. The germline clones are generated from the female adults (Parg27.1, FRT101/FRT101, ubi-GFP; hs-FLP38/+) after heat shock.Pargmutant germline clones are shown by the absence of GFP expression (green); F-actin is stained with phalloidin to visualize the cell membrane, and the oocyte is labelled with anti-orb antibody (blue). (f)Pargmutant follicle cell clones showing the normal localization of the oocyte in the posterior. The follicle cell clones are generated from the female adults (Parg27.1, FRT101/FRT101, ubi-GFP; en-Gal4,UAS-FLP38/+).Pargmutant follicle cell clones are shown by the absence of GFP expression (green). F-actin is stained with phalloidin to visualize the cell membrane. Arrow indicates the oocyte shown by the enrichment of F-actin in the ring canal. (g)Pargmutant germline and follicle cell clones in the anterior (white arrow). (h)Pargmutant clones, including germline and follicle cells, showing mislocalization of the oocyte in the lateral (red arrow). (g,h)Pargmutant germline and follicle cell clones are generated from the female adults (Parg27.1,FRT101/FRT101,ubi-GFP; hs-FLP38/+) after heat shock and shown by the absence of GFP expression (green), and the oocyte is labelled with anti-orb antibody (red). Scale bars,a,b,gandh, 10 μm;c-f, 20 μm. Figure 2: Parg expression in the ovary and mislocalization of the oocyte caused by Parg mutant clones. The anterior pole of all egg chambers is to the left, and the posterior pole is to the right. ( a ) Parg mRNA expression in the ovary of the wild type ( y,w ) detected by RNA in situ hybridization using Parg antisense probe. ( b ) The control of RNA in situ hybridization using Parg sense probe. ( c ) The expression of PARG-EGFP in the ovary induced by germline-specific GAL4 drivers. ( d ) The mock wild-type clones, including germline and polar follicle cells, showing the normal localization of the oocyte in the posterior. The oocyte is labelled with anti-orb antibody (red). The clones are generated from the female adults ( FRT101/FRT101, ubi-GFP; FLP38/+ ) after heat shock. ( e ) Parg mutant germline clones showing the normal localization of the oocyte in the posterior. The germline clones are generated from the female adults ( Parg 27.1 , FRT101/FRT101, ubi-GFP; hs-FLP38/+ ) after heat shock. Parg mutant germline clones are shown by the absence of GFP expression (green); F-actin is stained with phalloidin to visualize the cell membrane, and the oocyte is labelled with anti-orb antibody (blue). ( f ) Parg mutant follicle cell clones showing the normal localization of the oocyte in the posterior. The follicle cell clones are generated from the female adults ( Parg 27.1 , FRT101/FRT101, ubi-GFP; en-Gal4,UAS-FLP38/+ ). Parg mutant follicle cell clones are shown by the absence of GFP expression (green). F-actin is stained with phalloidin to visualize the cell membrane. Arrow indicates the oocyte shown by the enrichment of F-actin in the ring canal. ( g ) Parg mutant germline and follicle cell clones in the anterior (white arrow). ( h ) Parg mutant clones, including germline and follicle cells, showing mislocalization of the oocyte in the lateral (red arrow). ( g , h ) Parg mutant germline and follicle cell clones are generated from the female adults ( Parg 27.1 ,FRT101/FRT101,ubi-GFP; hs-FLP38/+ ) after heat shock and shown by the absence of GFP expression (green), and the oocyte is labelled with anti-orb antibody (red). Scale bars, a , b , g and h , 10 μm; c - f , 20 μm. Full size image The hrp38 mutants have reduced fertility To characterize the functions of the hrp38 gene during Drosophila development, we used one P-element insertion in exon 2 of the hrp38 gene ( w*,P[XP] d05172/ TM6B, Tb 1 ) [22] and a hrp38 region deficiency line ( w 1118 ; Df(3R) Exel6209 , P{XP-U} Exel6209 /TM6B, Tb 1 ) having a small deletion in exon 2 of the hrp38 gene [23] ( Supplementary Fig. S1a ). These mutations are lethal when homozygous. The hrp38 hemizygotes ( hrp38 d05172 / Df ) did not express hrp38 mRNA ( Supplementary Fig. S1b ), and had a significantly lower expression of Hrp38 protein than the wild type at the third-instar larvae stage ( Supplementary Fig. S1c ). In the complementation test, the P-element insertion ( hrp38 d05172 ) failed to complement the hrp38 deficiency ( Supplementary Table S1 ). Three-fourths of the hrp38 hemizygotes ( hrp38 d05172 / Df ; n =682) died before the pupal stage, indicating the importance of hrp38 for normal fly development. The incomplete penetrance may have proceeded from a partial overlap of hrp38 and hrp36 , whose functional domains are highly homologous [24] . hrp38 RNA interference (RNAi) lines (P{GD14939}v29523 and P{GD14939}v29524/CyO) were crossed with strains ubiquitously expressing GAL4 ( Act5C–GAL4 and tubP–GAL4 ). The results show that hrp38 RNAi causes lethality ( Supplementary Table S1 ). The expression of a UAS-Hrp38:RFP transgene induced by the ubiquitously expressed arm -GAL4 driver was sufficient to rescue lethality of the hemizygotes ( hrp38 d05172 /Df ) ( Supplementary Fig. S1d and Table S2 ). These results confirm that mutations of the hrp38 gene are fully responsible for lethality of the hemizygotes ( hrp38 d05172 /Df ). We observed that hemizygous female escapers had very low fertility (6 progeny per fly in the mutant versus 51 progeny per fly in the wild type after 5 days of crossing; n =100) and significantly reduced egg laying rates (0.1 egg per hour per fly versus 1.2 eggs per hour per fly, respectively), confirming that the hrp38 gene is required for oogenesis. The hrp38 gene regulates oocyte localization As the hrp38 mutants have reduced fertility, hrp38 functions during oogenesis were investigated. We observed that the Hrp38:GFP fusion protein in a protein trap line (ZCL588), in which GFP was spliced in the frame with the Hrp38-PE transcript [19] , was predominantly expressed in the nuclei of the somatic follicle cells and germline cells during all stages of oogenesis ( Fig. 3a,b ). As Hrp38:GFP expression is absent in the oocyte from stage 2 ( Fig. 3b ), it appears that Hrp38 expression is inhibited in the oocyte once the cyst moves down the germarium after the anterior–posterior axis is established. Therefore, we compared progression of oogenesis in the wild-type and hrp38 mutant. 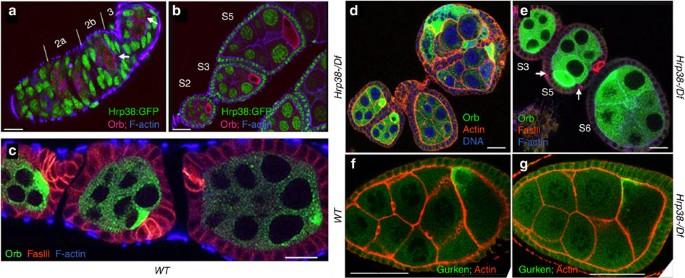Figure 3: Ovary developmental defects caused by thehrp38mutations. (a–e) Egg chambers stained with phalloidin to visualize filamentous actin in the cell membrane and anti-orb antibody to label the oocyte. The anterior pole of all the egg chambers is to the left, and the posterior pole is to the right. (a) The Hrp38:GFP expression pattern in the germarium. Arrows indicate the pre-oocytes in region 2b and the oocyte in region 3. (b) The Hrp38:GFP expression pattern in the stage 2, 3 and 5 egg chambers. (c) The wild type in which the oocyte is localized in the posterior pole. The egg chambers were stained with anti-FasIII (red) for labelling the polar cells. (d) Thehrp38hemizygotes showing the fused egg chambers. The egg chambers stained with Drag-5 (blue) to visualize DNA. (e) Thehrp38hemizygotes showing mislocalization of the oocytes. Arrows indicate the separated polar cells stained with anti-FasIII (red) in the lateral where the oocyte is localized in the stage 5 egg chamber. (f,g) Gurken protein localization in the oocytes of the wild type (f) and thehrp38mutant (g). Scale bars,a,b,dande, 10 μm;c, 20 μm;f,g, 30 μm. Figure 3: Ovary developmental defects caused by the hrp38 mutations. ( a – e ) Egg chambers stained with phalloidin to visualize filamentous actin in the cell membrane and anti-orb antibody to label the oocyte. The anterior pole of all the egg chambers is to the left, and the posterior pole is to the right. ( a ) The Hrp38:GFP expression pattern in the germarium. Arrows indicate the pre-oocytes in region 2b and the oocyte in region 3. ( b ) The Hrp38:GFP expression pattern in the stage 2, 3 and 5 egg chambers. ( c ) The wild type in which the oocyte is localized in the posterior pole. The egg chambers were stained with anti-FasIII (red) for labelling the polar cells. ( d ) The hrp38 hemizygotes showing the fused egg chambers. The egg chambers stained with Drag-5 (blue) to visualize DNA. ( e ) The hrp38 hemizygotes showing mislocalization of the oocytes. Arrows indicate the separated polar cells stained with anti-FasIII (red) in the lateral where the oocyte is localized in the stage 5 egg chamber. ( f , g ) Gurken protein localization in the oocytes of the wild type ( f ) and the hrp38 mutant ( g ). Scale bars, a , b , d and e , 10 μm; c , 20 μm; f , g , 30 μm. Full size image In a wild-type ovariole, all oocytes showing stronger Orb staining were positioned in the posterior pole adjacent to a pair of polar follicle cells stained with FasIII ( Fig. 3c ). hrp 38 mutant females displayed defects during egg development, including fused egg chambers (7%, n =125, Fig. 3d ) and mislocalization of the oocyte (11%, n =142, Fig. 3e ). Mispositioned oocytes in the hrp38 mutants were found either at the anterior pole ( Fig. 3e , S6 egg) or on the lateral side of the egg chamber ( Fig. 3e , S5 egg). In the S5 egg, a pair of polar cells was separated from each other instead of the usual connection in the poles ( Fig. 3e , S5 egg), suggesting that Hrp38 is involved in defining the follicle cell patterns. The wild-type strain showed none of these defects ( n =135; Fig. 3c ). Expression of a UASp-hrp38:RFP transgene in the germline cells fully rescued the defective phenotypes of the hrp38 hemizygotes ( hrp38 d05172 /Df ; n =216, Supplementary Fig. S2a,b ), confirming that hrp38 loss-of-function mutation is responsible for the observed phenotypes. Although Hrp38 function is necessary for tissue polarity and oocyte positioning ( Fig. 3d,e ), this protein was not required for asymmetric localization of cytoplasmic markers such as Gurken ( Fig. 3f,g ). According to this last observation, Hrp38 controls tissue polarization by regulating extracellular interaction rather than polarization of cytoplasm within cells. Parg and Hrp38 control DE-cadherin-dependent oocyte localization It is well known that the posterior localization of the oocyte requires cadherin-dependent adhesion between the follicle cells surrounding the posterior pole and the oocyte [9] , [10] . As reported previously [9] , DE-cadherin concentration in wild-type ovaries is considerably greater at the interface between the oocyte and posterior follicle cells than between nurse cells and anterior follicle cells ( Fig. 4a ). In hrp38 mutant egg chambers, DE-cadherin expression was the highest at the anterior part of the egg chamber, a condition resulting in mislocalization of the oocyte to the anterior end ( Fig. 4b , green arrow). The hrp38 mutant had lower expression of DE-cadherin at the AJs of the lateral follicle cells ( Fig. 4b , yellow arrow) relative to the wild type ( Fig. 4a , yellow arrow). The altered expression of DE-cadherin was shown in 20% of hrp38−/− mutant egg chambers ( n =130), among which 75% had relatively higher expression in the anterior than in the posterior pole, whereas 25% had no accumulation. All these egg chambers displayed either oocyte mislocalization or fused egg chambers. Immunoblotting analysis showed that DE-cadherin expression in the hrp38 mutant ovary was approximately threefold decreased relative to the wild-type ovary ( Supplementary Fig. S3a ). Germline expression of the UASp-hrp38:RFP transgene restored the normal expression pattern of DE-cadherin in the hrp38 mutant egg chambers ( n =90; Supplementary Fig. S2c ), confirming that hrp38 loss-of-function causes decreased DE-cadherin expression in the ovary. 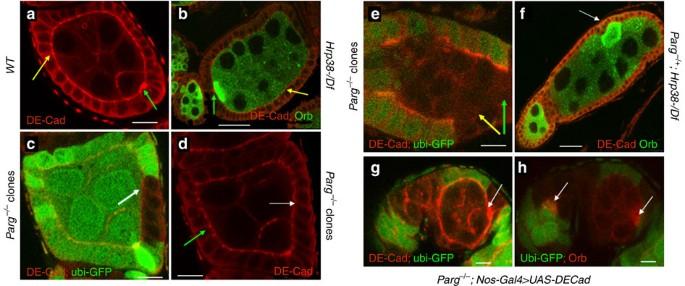Figure 4: Regulation of DE-cadherin expression by pADPr modification of Hrp38. The anterior pole of all the egg chambers is to the left, and the posterior pole is to the right. (a) DE-cadherin expression in the egg chamber of the wild type. (b) DE-cadherin expression in the egg chambers of thehrp38mutant. The oocytes were labelled with anti-orb antibody. Inaandb, green arrow indicates the interface between oocyte and polar cells, and yellow arrow indicates the adherens junctions between the lateral follicle cells. (c) DE-cadherin expression inPargfollicle cell clones.Pargmutant follicle cell clones are shown by the absence of GFP expression. (d) DE-cadherin expression in the wild-type (green arrow) andPargfollicle cell clones (white arrow) as inc. Arrows inc,dindicate the adherens junctions between the lateral follicle cells. (e) DE-cadherin expression inParggermline and follicle cell clones.Pargmutant germline and follicle cell clones are shown by the absence of GFP expression (green). Green arrow indicates the interface between germline cells and posterior follicle cells, and yellow arrow indicates the adherens junctions between the lateral follicle cells. (f) DE-cadherin expression in the egg chambers of the genotype (Parg−/+;hrp38d05172/Df). The oocyte (white arrow) is labelled with anti-orb antibody. (g,h) Expression of DE-cadherin in the germline rescued oocyte mislocalization inPargmutant clones. The full genotype is:Parg27.1, FRT101/Ubi-GFP, FRT101; FLP38/Nos-Gal4; UASp-DEcadherin/+. (g) The elevated DE-cadherin expression (white arrow) in the posterior pole of one egg chamber with thePargmutant germline and follicle cell clones, including the polar cells. (h) The normal oocyte localization (white arrow) in the same egg chamber as ing. The oocyte is labelled with anti-orb antibody (red). Scale bars,a–f, 10 μm;g,h, 5 μm. Figure 4: Regulation of DE-cadherin expression by pADPr modification of Hrp38. The anterior pole of all the egg chambers is to the left, and the posterior pole is to the right. ( a ) DE-cadherin expression in the egg chamber of the wild type. ( b ) DE-cadherin expression in the egg chambers of the hrp38 mutant. The oocytes were labelled with anti-orb antibody. In a and b , green arrow indicates the interface between oocyte and polar cells, and yellow arrow indicates the adherens junctions between the lateral follicle cells. ( c ) DE-cadherin expression in Parg follicle cell clones. Parg mutant follicle cell clones are shown by the absence of GFP expression. ( d ) DE-cadherin expression in the wild-type (green arrow) and Parg follicle cell clones (white arrow) as in c . Arrows in c , d indicate the adherens junctions between the lateral follicle cells. ( e ) DE-cadherin expression in Parg germline and follicle cell clones. Parg mutant germline and follicle cell clones are shown by the absence of GFP expression (green). Green arrow indicates the interface between germline cells and posterior follicle cells, and yellow arrow indicates the adherens junctions between the lateral follicle cells. ( f ) DE-cadherin expression in the egg chambers of the genotype ( Parg− /+; hrp38 d05172 /Df ). The oocyte (white arrow) is labelled with anti-orb antibody. ( g , h ) Expression of DE-cadherin in the germline rescued oocyte mislocalization in Parg mutant clones. The full genotype is: Parg 27.1 , FRT101/Ubi-GFP, FRT101; FLP38/Nos-Gal4; UASp-DEcadherin/+ . ( g ) The elevated DE-cadherin expression (white arrow) in the posterior pole of one egg chamber with the Parg mutant germline and follicle cell clones, including the polar cells. ( h ) The normal oocyte localization (white arrow) in the same egg chamber as in g . The oocyte is labelled with anti-orb antibody (red). Scale bars, a – f , 10 μm; g , h , 5 μm. Full size image To test whether reduced expression of DE-cadherin is responsible for oocyte mislocalization in the hrp38 mutants, we cloned the DE-cadherin coding region without its 5′-untranslated region (UTR) into pUASp vector and used nos-GAL4 to drive expression of the transgene in germline cells in the hrp38 mutant background ( Supplementary Fig. S3a ). DE-cadherin expression in the germline cells was sufficient to restore normal oocyte localization in the hrp38 mutants ( n =112; Supplementary Fig. S3b,c ). After expressing DE-cadherin transgene in the germline cells, we did not observe any phenotypes exhibited by the hrp38 mutant ( n =136, Supplementary Fig. S3d,e ). This finding shows that proper oocyte polarity established by DE-cadherin-mediated AJs in the germarium also affects the fate of stalk and polar follicle cells in the later stages of oogenesis. Taken together, these results suggest that decreased DE-cadherin expression in the germline cells is the underlying cause for the observed phenotypes in the hrp38 mutant. Consistent with oocyte mislocalization observed in Parg mutant follicle and germline cell clones ( Fig. 2g,h ), the loss of Parg in both germ cells and polar cells led to loss of DE-cadherin expression (compare Fig. 4c with e). Expression of a pUASp-DE-cadherin transgene without its 5′UTR in the germline cell using nos-Gal4 driver was sufficient to rescue the oocyte mislocalization in the Parg mutant follicle, including the polar cells and germline cell clones ( n =34, Fig. 4g,h ). Therefore, loss of DE-cadherin expression is responsible for oocyte mislocalization in Parg mutant clones. These results show that the hrp38 and Parg genes regulate the expression of DE-cadherin, required for proper oocyte positioning. As Hrp38 shows greater association with pADPr in the Parg mutant than in the wild type [19] , we proposed that pADPr binding to Hrp38 regulates DE-cadherin expression. To test this hypothesis, we removed one copy of the Parg gene in the hrp38 mutant background ( Parg− /+; hrp d05172 /Df ). The mutant genotype ( Parg− /+; hrp d05172 /Df ) had an increased proportion of mislocalized oocytes relative to the hrp38 mutant alone (19% versus 11%, respectively, n =176; t -test P <0.05). Most of the mislocalized oocytes in the genotype ( Parg− /+; hrp d05172 /Df ) showed no accumulation of DE-cadherin in either pole, resulting in laterally positioned oocytes ( Fig. 4f , arrow), which resembled the phenotypes caused by DE-cadherin null mutation [10] . Expression of Hrp38:RFP ( n =152) or DE-cadherin transgene ( n =165) in the germline fully rescued oocyte mislocalization in ( Parg− /+; hrp d05172 /Df ). Hrp38 controls GSC maintenance Besides oocyte localization, DE-cadherin is required for GSC maintenance by anchoring GSCs within the niche through AJs [6] ( Fig. 5a ). If controlling DE-cadherin levels is a general function of pADPr binding to Hrp38, hrp38 and Parg mutants should display defects in DE-cadherin-mediated regulation of GSCs. Indeed, we found that Hrp38:GFP is expressed in GSCs, as well as in cap cells of the GSC niche ( Fig. 5b ). Similar to the wild type (n=85), most germaria of hrp38 mutants had two or three GSCs at day 3 after eclosion ( n =82) ( Supplementary Fig. S4a ). At day 10, wild-type germaria had two or three GSCs ( n =94; Fig. 5c ), although most germaria in the hrp38 mutant (72%) had only one GSC left ( n =91; Fig. 5d and Supplementary Fig. S4a ). At 17 days after eclosion, 70% of germaria in the hrp38 mutants had lost their GSCs ( n =96; Fig. 5e,f and Supplementary Fig. S4a ), whereas the wild type still retained GSC self-renewal ability ( n =90; Fig. 5f ). The expression of the hrp38:RFP transgene in the germline cells restored GSC self-renewal ability of the hrp38 mutant ( Fig. 5f , Supplementary Fig. S4a,b ), confirming that the hrp38 gene is required for GSC maintenance. 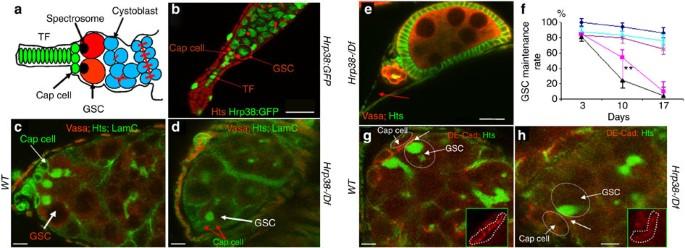Figure 5: Thehrp38gene is required for maintenance of germline stem cells. (a) Simplified diagram of the germarium structure. GSCs having the round spectrosome are localized in the niche containing terminal filament (TF) and cap cells. The cystoblast and its progeny are interconnected through the ring canals. (b) Thehrp38expression in GSC and cap cells in the tip of germarium of the Hrp38:GFP strain. GSC is labelled with anti-hts antibody for spectrosome (red). (c) Ten-day-old germarial tip of the wild type. (d) Ten-day-old germarial tip of thehrp38mutant. Incandd, GSCs are labelled with anti-hts (green) and anti-Vasa antibody (red). The cap cells are labelled with anti-Lam-C antibody (green). (e) Seventeen-day-old germarium of thehrp38mutant showing the last egg chamber. The fusome in the last egg chamber is shown as yellow after labelling with anti-hts (green) and anti-Vasa antibody (red). Arrow indicates an empty germarium. (f) Graph showing GSC maintenance rate of the indicated genotypes. The GSC maintenance rate was based on the percent of the germaria with two to three GSCs at the indicated time after eclosion. Two germaria with one GSC was counted as one wild-type germarium to calculate their maintenance rate. Symbols: dark blue line with diamonds (the wild type;n=85); pink line with squares (hrp38−/−;n=82); black line with triangles (Parg+/−;hrp38−/−;n=80); light blue with crosses (RFP:Hrp38/nos-Gal4;hrp38−/−;n=92); dark magenta line with stars (DE-cad/nos-Gal4; hrp38−/−;n=110). The error bar represents the standard deviation of the proportion normalized with the sample size. **P<0.01, analysed byt-test. (g) DE-cadherin expression in the 10-day-old GSC in the wild type. (h) DE-cadherin expression in the 10-day-old GSCs in thehrp38mutant. Ingandh, GSCs are labelled with anti-hts (green). Insets showed DE-cadherin expression in the interface (arrows) between GSC and the cap cells (circled). Scale bars,b,e, 10 μm;c,d,g,h, 5 μm. Figure 5: The hrp38 gene is required for maintenance of germline stem cells. ( a ) Simplified diagram of the germarium structure. GSCs having the round spectrosome are localized in the niche containing terminal filament (TF) and cap cells. The cystoblast and its progeny are interconnected through the ring canals. ( b ) The hrp38 expression in GSC and cap cells in the tip of germarium of the Hrp38:GFP strain. GSC is labelled with anti-hts antibody for spectrosome (red). ( c ) Ten-day-old germarial tip of the wild type. ( d ) Ten-day-old germarial tip of the hrp38 mutant. In c and d , GSCs are labelled with anti-hts (green) and anti-Vasa antibody (red). The cap cells are labelled with anti-Lam-C antibody (green). ( e ) Seventeen-day-old germarium of the hrp38 mutant showing the last egg chamber. The fusome in the last egg chamber is shown as yellow after labelling with anti-hts (green) and anti-Vasa antibody (red). Arrow indicates an empty germarium. ( f ) Graph showing GSC maintenance rate of the indicated genotypes. The GSC maintenance rate was based on the percent of the germaria with two to three GSCs at the indicated time after eclosion. Two germaria with one GSC was counted as one wild-type germarium to calculate their maintenance rate. Symbols: dark blue line with diamonds (the wild type; n =85); pink line with squares ( hrp38−/− ; n =82); black line with triangles ( Parg+/− ; hrp38−/− ; n =80); light blue with crosses ( RFP:Hrp38/nos-Gal4 ; hrp38−/− ; n =92); dark magenta line with stars ( DE-cad/nos-Gal4 ; hrp38 − / − ; n =110). The error bar represents the standard deviation of the proportion normalized with the sample size. ** P <0.01, analysed by t -test. ( g ) DE-cadherin expression in the 10-day-old GSC in the wild type. ( h ) DE-cadherin expression in the 10-day-old GSCs in the hrp38 mutant. In g and h , GSCs are labelled with anti-hts (green). Insets showed DE-cadherin expression in the interface (arrows) between GSC and the cap cells (circled). Scale bars, b , e , 10 μm; c , d , g , h , 5 μm. Full size image DE-cadherin is strongly expressed in the interface between GSCs and cap cells in the wild-type fly [6] for anchoring the GSC within the niche ( Fig. 5g ). We examined DE-cadherin expression in 10-day-old wild-type and hrp38 mutant GSCs ( Fig. 5g,h ). DE-cadherin expression level at the interface between the cap cells and the one remaining GSC in 10-day-old hrp38 mutants was reduced by 70%, relative to that in the wild type ( n =10, Fig. 5h ). Normal expression levels of DE-cadherin in the interface between cap cells and GSC were restored by expressing UASp-hrp38:RFP transgene in GSCs in 14-day-old hrp38 mutants ( n =128, Supplementary Fig. S4c ). Ectopic expression of DE-cadherin in the germline significantly increased the GSC self-renewal ability in the hrp38 mutant background ( Figs 5f , Supplementary Fig. S4d–f ), confirming that decreased DE-cadherin expression causes the loss of GSC self-renewal ability in the hrp38 mutants. To maintain their undifferentiated state, GSCs must maintain low levels of the Bag-of-marbles (BAM) differentiation factor [25] , [26] , [27] . Compared with the wild-type fly ( n =54, Supplementary Fig. S5a ), BAM was not prematurely expressed in the hrp38 mutant GSCs ( n =58, Supplementary Fig. S5b ). Using anti-cleaved Caspase-3 antibody, which has been used successfully to detect apoptosis in the Drosophila Lsd1 mutant GSC [28] , no strong apoptosis signals were detected in the GSC of 10-day-old hrp38 mutants ( n =58, Supplementary Fig. S5b ). These observations largely exclude the possibility that either premature differentiation of GSC through the BAM-dependent pathway or apoptosis caused the loss of GSC maintenance in the hrp38 mutant. Parg controls DE-cadherin-dependent stem cell maintenance Because Parg mutant germline cell and follicle cell clones lost the expression of DE-cadherin ( Fig. 4e ), we investigated whether Parg is required for GSC self-renewal. We found that Parg mRNA and PARG-EGFP are expressed in the wild-type GSCs ( Fig. 6a and Supplementary Fig. S5c ) and by germline-specific GAL4 driver ( Fig. 6b ). To determine whether Parg is required for GSC self-renewal, we used a FLP/FRT recombination system to generate negatively labelled Parg mutant GSCs, which were identified by the absence of GFP expression ( Fig. 6c,d ). The loss rates of the mutant GSCs were computed based on a published procedure [6] . Three days after clone induction, Parg mutant GSCs and cysts were present in the germarium ( n =53; Fig. 6c ). Two weeks after clone induction, Parg mutant GSCs were lost in 95% of the germaria ( n =58, Supplementary Fig. S5d ) where the developing Parg mutant egg chamber was visible ( Fig. 6d ). Marked wild-type GSCs were still retained in 80% of germaria ( n =56, Supplementary Fig. S5d ). Therefore, we conclude that Parg is required for maintaining GSCs and infer that poly(ADP-ribosyl)ation strongly affects GSC maintenance. 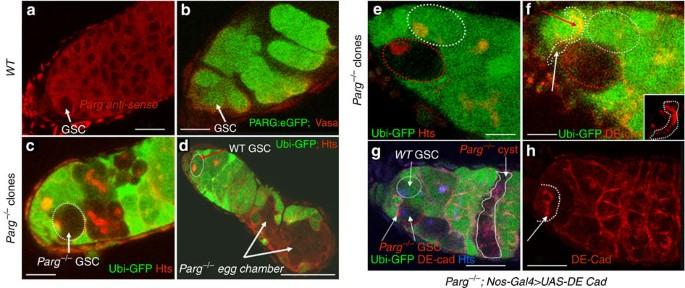Figure 6: Loss of DE-cadherin expression inPargmutant GSC. (a)PargmRNA expression in GSC in the wild type (y,w), as detected by RNAin situhybridization usingPargantisense probe. (b) The expression of PARG-EGFP in GSCs by germline-specific GAL4 drivers. (c) Germaria showing a 3-day-oldPargmutant GSC with loss of GFP expression. GSC is labelled with anti-hts (red). (d) 17-day-old germarium showing the loss ofPargmutant GSC. The loss ofPargmutant GSC was shown by the presence of two mutant egg chambers. GSC labelled with anti-hts antibody (red). (e,f) DE-cadherin expression in a germarium tip carrying one wild-type GSC and onePargmutant GSC 1 week after clone induction. White circle: the wild-type GSC (GFP positive); Red cycle:Pargmutant GSC (GFP-negative); GSCs are labelled with anti-hts antibody ine. Inset infshows DE-cadherin expression in the interface between GSCs and wild-type cap cells (arrow indicated inf). (g) 17-day-old germarium showingPargmutant GSC and its progeny. (h) Expression of DE-cadherin in the germline cells rescuedPargmutant GSC loss as shown ing. The full genotype (gandh):Parg27.1, FRT101/Ubi-GFP, FRT101; FLP38/Nos-Gal4; UASp-DEcadherin/+. GSC labelled with anti-hts antibody (blue). Arrows ingandhindicate DE-cadherin expression in the interface between GSCs and wild-type cap cells. Scale bars,a–c,e–h, 10 μm;d, 20 μm. Figure 6: Loss of DE-cadherin expression in Parg mutant GSC. ( a ) Parg mRNA expression in GSC in the wild type (y,w), as detected by RNA in situ hybridization using Parg antisense probe. ( b ) The expression of PARG-EGFP in GSCs by germline-specific GAL4 drivers. ( c ) Germaria showing a 3-day-old Parg mutant GSC with loss of GFP expression. GSC is labelled with anti-hts (red). ( d ) 17-day-old germarium showing the loss of Parg mutant GSC. The loss of Parg mutant GSC was shown by the presence of two mutant egg chambers. GSC labelled with anti-hts antibody (red). ( e , f ) DE-cadherin expression in a germarium tip carrying one wild-type GSC and one Parg mutant GSC 1 week after clone induction. White circle: the wild-type GSC (GFP positive); Red cycle: Parg mutant GSC (GFP-negative); GSCs are labelled with anti-hts antibody in e . Inset in f shows DE-cadherin expression in the interface between GSCs and wild-type cap cells (arrow indicated in f ). ( g ) 17-day-old germarium showing Parg mutant GSC and its progeny. ( h ) Expression of DE-cadherin in the germline cells rescued Parg mutant GSC loss as shown in g . The full genotype ( g and h ): Parg 27.1 , FRT101/Ubi-GFP, FRT101; FLP38/Nos-Gal4; UASp-DEcadherin/+ . GSC labelled with anti-hts antibody (blue). Arrows in g and h indicate DE-cadherin expression in the interface between GSCs and wild-type cap cells. Scale bars, a – c , e – h , 10 μm; d , 20 μm. Full size image To test whether the hrp38 and Parg genes interact to control GSC maintenance, we assessed the changes in number of GSCs in ( Parg− /+; hrp d05172 /Df ) genotype with aging. Removing one copy of the Parg gene caused a more rapid GSC loss in the hrp38 mutant ( Fig. 5f and Supplementary Fig. S4a ). Expression of Hrp38:RFP or DE-cadherin transgenes in the germline fully restored GSC maintenance ability ( Parg− /+; hrp d05172 /Df ; Supplementary Fig. S4a ). These results demonstrate that genetic interaction between the hrp38 and Parg genes controls GSC maintenance. Further, we examined DE-cadherin expression in Parg mutant GSC clones 1 week after clone induction. DE-cadherin accumulated in the interface between the wild-type GSC (GFP-positive) and wild-type cap cells, yet its expression was fourfold reduced in Parg mutant GSC clones (GFP-negative) when compared with DE-cadherin accumulation in wild-type GSC cells ( Fig. 6e,f ; n =10). With expression of the DE-cadherin transgene in the germline cells ( Fig. 6g,h ), the Parg mutant GSCs were still maintained in 65% of germaria ( n =70) 2 weeks after clone induction, which is comparable to the maintenance rate of the marked wild-type GSCs ( Supplementary Fig. S5d ). Therefore, the loss of DE-cadherin expression, resulting in the failure to strongly anchor the Parg mutant GSC within the niche by AJs, likely explains the Parg mutant's loss of GSC self-renewal. Similar to hrp38 mutant GSCs, Parg mutant GSCs were lost neither by apoptosis ( Supplementary Fig. S5e,f ) nor by inappropriate expression of Bam ( Supplementary Fig. S5g,h ). pADPr inhibits Hrp38-dependent DE-cadherin translation To further evaluate how pADPr binding to Hrp38 controls DE-cadherin expression, we examined mRNA and protein expression levels of DE-cadherin in the hrp38 and Parg mutants at the third-instar larval stage. No significant difference in mRNA expression levels was found between the wild-type and the hrp38 mutant or the Parg mutant by quantitative reverse transcription-PCR ( Supplementary Methods ; Fig. 7a ), suggesting that pADPr binding to Hrp38 does not affect DE-cadherin transcription. Although the DE-cadherin gene has only one transcript with a constitutively spliced intron (Flybase), we examined potential effects of hrp38 or Parg mutation on splicing of DE-cadherin transcript. Splicing defects were not observed in hrp38 and Parg mutants, suggesting that Hrp38 and its association with pADPr do not regulate DE-cadherin by affecting splicing. Immunoblotting analysis ( Supplementary Methods ) showed that protein expression levels of DE-cadherin in hrp38 and Parg mutants was decreased by 3.5- and 4.0-fold, respectively, relative to the wild-type ( Fig. 7b ), suggesting that the association of Hrp38 with pADPr regulates DE-cadherin expression at the translational level. 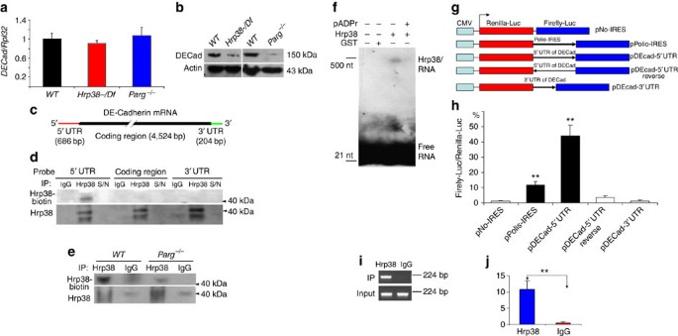Figure 7: pADPr disrupts Hrp38 binding to 5′UTR of DE-cadherin conferring IRES activity. (a) The mRNA expression level of DE-cadherin in the different genotypes at the wandering third-instar larvae stage. (b) The protein expression level of DE-cadherin in the different genotypes at the wandering third-instar larvae stage. (c) The structure of DE-cadherin transcript. The biotin-labelled probes were made from three regions (5′UTR, coding region and 3′UTR). (d) Hrp38 binding to 5′UTR of DE-cadherin in the ovary is shown by ultraviolet crosslinking analysis. The ovarian lysate from the wild-type fly (y,w)crosslinked to the biotin-labelled RNA probes as indicated was IPed with rabbit anti-Hrp38 antibody or normal rabbit IgG as the control for IP. The supernatant (S/N), which was obtained after each IP, was run in the same blot to show the efficiency of RNase treatment. (e) Decreased amounts of Hrp38 protein binding to 5′UTR of DE-cadherin in thePargmutant. Indande, Hrp38 protein binding to biotin-labelled RNA probe was detected with Streptavidin. The same blot was stripped and probed with anti-Hrp38 antibody to show IP efficiency. (f) Inhibition of Hrp38 binding to its target RNA motif by poly(ADP-ribose). The biotin-labelled G-rich RNA element (5′-CAGGGCGCGCACUGUACGAG-3′) within 5′UTR of DE-cadherin was incubated with the components as indicated. (g) Diagrams of the different constructs for dual luciferase assay. CMV: cytomegalovirus (CMV) promoter; pNO-IRES (negtative control); pPolio-IRES (positive control); pDEcad 5′UTR:DE-cadherin5′UTR cloned into the vector in the forward orientation. pDEcad 5′UTR-reverse (spacer control); pDEcad-3′UTR (element control). (h) The ratio of firefly-to-Renilla luciferase activity after the transfection of the different constructs as indicated intoDrosophilaS2 cells. (i,j) The association of Hrp38 with the transcript from pDEcad 5′UTR-luciferase construct shown by regular reverse transcription (RT)-PCR (i) and quantitative RT-PCR (j) after RNA-IP. RNA-IP was done using anti-Hrp38 antibody or rabbit IgG as a control after the transfection of pDEcad-5′UTR construct into S2 cells. The error bars ina,handjrepresents the standard deviation from three independent experiments. **P<0.01, analysed byt-test. Figure 7: pADPr disrupts Hrp38 binding to 5′UTR of DE-cadherin conferring IRES activity. ( a ) The mRNA expression level of DE-cadherin in the different genotypes at the wandering third-instar larvae stage. ( b ) The protein expression level of DE-cadherin in the different genotypes at the wandering third-instar larvae stage. ( c ) The structure of DE-cadherin transcript. The biotin-labelled probes were made from three regions (5′UTR, coding region and 3′UTR). ( d ) Hrp38 binding to 5′UTR of DE-cadherin in the ovary is shown by ultraviolet crosslinking analysis. The ovarian lysate from the wild-type fly ( y,w) crosslinked to the biotin-labelled RNA probes as indicated was IPed with rabbit anti-Hrp38 antibody or normal rabbit IgG as the control for IP. The supernatant (S/N), which was obtained after each IP, was run in the same blot to show the efficiency of RNase treatment. ( e ) Decreased amounts of Hrp38 protein binding to 5′UTR of DE-cadherin in the Parg mutant. In d and e , Hrp38 protein binding to biotin-labelled RNA probe was detected with Streptavidin. The same blot was stripped and probed with anti-Hrp38 antibody to show IP efficiency. ( f ) Inhibition of Hrp38 binding to its target RNA motif by poly(ADP-ribose). The biotin-labelled G-rich RNA element (5′-CAGGGCGCGCACUGUACGAG-3′) within 5′UTR of DE-cadherin was incubated with the components as indicated. ( g ) Diagrams of the different constructs for dual luciferase assay. CMV: cytomegalovirus (CMV) promoter; pNO-IRES (negtative control); pPolio-IRES (positive control); pDEcad 5′UTR: DE-cadherin 5′UTR cloned into the vector in the forward orientation. pDEcad 5′UTR-reverse (spacer control); pDEcad-3′UTR (element control). ( h ) The ratio of firefly-to-Renilla luciferase activity after the transfection of the different constructs as indicated into Drosophila S2 cells. ( i , j ) The association of Hrp38 with the transcript from pDEcad 5′UTR-luciferase construct shown by regular reverse transcription (RT)-PCR ( i ) and quantitative RT-PCR ( j ) after RNA-IP. RNA-IP was done using anti-Hrp38 antibody or rabbit IgG as a control after the transfection of pDEcad-5′UTR construct into S2 cells. The error bars in a , h and j represents the standard deviation from three independent experiments. ** P <0.01, analysed by t -test. Full size image Next, we tested whether Hrp38 protein could bind to DE-cadherin mRNA directly in the ovary. Using ultraviolet crosslinking, biotin-labelled probes were made from three distinct regions (5′UTR, coding region and 3′UTR) of DE-cadherin ( Fig. 7c ). Ultraviolet crosslinking experiments showed that Hrp38 binds only to the 5′UTR of DE-cadherin mRNA in wild-type ovaries ( Fig. 7d ). Association of Hrp38 with DE-cadherin transcripts was further verified by in vivo RNA immunoprecipitation (IP; Supplementary Methods ) using anti-Hrp38 antibody in the Drosophila ovary ( Supplementary Fig. S6a,b ). Our previous study demonstrated that pADPr binding to Hrp38 reduced ability of this protein to bind RNA [19] . In humans, pADPr modification is known to inhibit the RNA-binding ability of hnRNP A1 [19] , the mammalian homologue of Hrp38 (ref. 29 ). To assess the role of Hrp38 modification by pADPr in Drosophila , we tested whether poly(ADP-ribosyl)ation could inhibit Hrp38 binding to the 5′UTR of DE-cadherin using ultraviolet crosslinking. Total protein was extracted from wild-type or Parg mutant third-instar larvae and was crosslinked to the 5′UTR of DE-cadherin. The amount of Hrp38 protein binding to the 5′UTR of DE-cadherin was 3.8-fold decreased in the Parg mutant, relative to that in the wild-type, suggesting that association with pADPr inhibits Hrp38 binding to the 5′UTR of DE-cadherin ( Fig. 7e ). Based on the finding that human hnRNPA1 has the strongest binding affinity to the G-rich RNA element (5′-UAUGAUAGGGACUUAGGGUG-3′) [30] , a potential binding site of Hrp38 (413-5′-CAGGGCGCGCACUGUACGAG-3′-432 bp) was identified within the DE-cadherin 5′UTR region. To test whether Hrp38 could bind to this G-rich motif, Hrp38 proteins were generated and purified ( Supplementary Fig. S6c ). The dot-blot assay confirmed that pADPr binds to Hrp38 protein in vitro ( Supplementary Fig. S6d ). An electrophoretic mobility shift assay showed that Hrp38 binds to this RNA motif ( Fig. 7f , lane 3). Pre-incubation of Hrp38 protein with pADPr almost completely abolished Hrp38 binding to this RNA motif ( Fig. 7f , lane 4). This result confirms that pADPr strongly inhibits the interaction between Hrp38 and RNA in vitro and provides additional evidence that association with pADPr inhibits Hrp38 binding to the 5′UTR of DE-cadherin. Hrp38 is required for IRES-dependent DE-cadherin translation The 5′UTR (686 bp) of DE-cadherin is much longer than the average size of 256 bp in 5′UTR of Drosophila genes [31] , implying that the DE-cadherin 5′UTR may have the ability to initiate an internal ribosome entry site (IRES)-mediated translation. Nucleotide sequence of IRES allows translation initiation in the middle of an mRNA sequence [32] . To test whether Hrp38 binding to the DE-cadherin 5′UTR promotes IRES-dependent translation, the 5′UTR of DE-cadherin was cloned into the upstream sequence of the firefly luciferase gene in Renilla/Firefly luciferase reporter plasmid ( Fig. 7g ). After transfection into Drosophila S2 cells, firefly and Renilla luciferase activities were measured. As a positive control, the Poliovirus IRES showed tenfold increase of luciferase activity relative to the control construct (pNo-IRES; Fig. 7h ). In contrast, the luciferase activity in cells transfected with DE-cadherin 5′UTR construct (p5′UTR DE-cad) was increased 40-fold, relative to the control construct ( Fig. 7h ). The efficient induction of IRES-mediated translation by the DE-cadherin 5′UTR is similar to that found in the 5′UTRs of other genes in Drosophila [33] . Neither the DE-cadherin 5′UTR in reverse orientation, as a spacer control, nor DE-cadherin 3′UTR, as an element control, show a significant increase in firefly luciferase activity, relative to the control ( Fig. 7h ). Consequently, the DE-cadherin 5′UTR has a strong ability to induce IRES-mediated translation. Furthermore, in vivo RNA IP showed that Hrp38 was associated with the transcript from DE-cadherin -5′UTR luciferase construct after transfection into Drosophila S2 cells ( Fig. 7i–j ), suggesting that Hrp38 is an IRES transacting factor for promoting cap-independent translation of DE-cadherin mRNA. Our experimental findings suggest that pADPr binding to Drosophila hnRNPA1 homologue Hrp38 regulates stem cell maintenance and oocyte polarity ( Fig. 8a–c ). Earlier research demonstrated that Hrp38 regulates alternative splicing [19] , [34] , whereas hnRNPA1 was reported to control translation initiation through an IRES-mediated mechanism by binding to the 5′UTR of regulated genes [35] , [36] . Here we show that pADPr association with Hrp38 controls DE-cadherin translation through an IRES-mediated mechanism. As Hrp38 binds to the 5′UTR of DE-cadherin and is associated with the DE-cadherin 5′UTR-luciferase transcript, it seems very likely that Hrp38 is an IRES transacting factor for promoting DE-cadherin translation. In mammals, post-translational modification of hnRNPA1 has been shown to regulate IRES-dependent translation. For instance, phosphorylation of hnRNPA1 can promote the binding of hnRNPA1 to IRES of c- Myc in myeloma cells [37] . Similarly, our results suggest that pADPr modification of hnRNPs negatively regulates IRES-mediated translation by inhibiting the binding of hnRNPs to IRES. 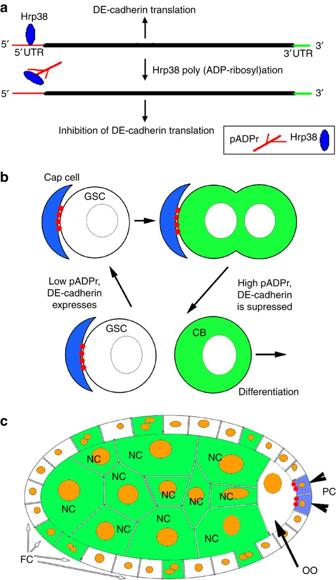Figure 8: Hrp38 modification by pADPr controls maintenance of GSC and oocyte localization. (a) pADPr binding to Hrp38 regulates DE-cadherin translation. Hrp38 binds to 5′UTR of DE-cadherin to promote translation by IRES-mediated manner. Once Hrp38 is modified with pADPr and dissociated from 5′UTR of DE-cadherin, its translation is inhibited. (b) pADPr modification of Hrp38 regulates DE-cadherin translation for germline stem cell (GSC) maintenance. DE-cadherin (red) accumulates in the interface between cap cells and GSC, keeping GSC in the stem cell niche. High level of pADPr (green) during mitosis and in cystoblasts suppresses translation of DE-cadherin. Suppression of DE-cadherin production promotes cystoblasts to leave stem cell niche and differentiate. (c) pADPr binding to Hrp38 regulates DE-cadherin translation for oocyte (OO) localization in maturating egg chamber. Low level of pADPr in the oocyte and mitotically quiescent polar cells (PC) allows translating DE-cadherin (red) and positioning the oocyte in the posterior pole of the egg chamber. High level of pADPr (green) in nurse cells and mid-body follicle cells inhibits translation of DE-cadherin. FC, follicle cells. Figure 8: Hrp38 modification by pADPr controls maintenance of GSC and oocyte localization. ( a ) pADPr binding to Hrp38 regulates DE-cadherin translation. Hrp38 binds to 5′UTR of DE-cadherin to promote translation by IRES-mediated manner. Once Hrp38 is modified with pADPr and dissociated from 5′UTR of DE-cadherin, its translation is inhibited. ( b ) pADPr modification of Hrp38 regulates DE-cadherin translation for germline stem cell (GSC) maintenance. DE-cadherin (red) accumulates in the interface between cap cells and GSC, keeping GSC in the stem cell niche. High level of pADPr (green) during mitosis and in cystoblasts suppresses translation of DE-cadherin. Suppression of DE-cadherin production promotes cystoblasts to leave stem cell niche and differentiate. ( c ) pADPr binding to Hrp38 regulates DE-cadherin translation for oocyte (OO) localization in maturating egg chamber. Low level of pADPr in the oocyte and mitotically quiescent polar cells (PC) allows translating DE-cadherin (red) and positioning the oocyte in the posterior pole of the egg chamber. High level of pADPr (green) in nurse cells and mid-body follicle cells inhibits translation of DE-cadherin. FC, follicle cells. Full size image The inhibitory function of pADPr binding to hnRNPs likely occurs in the nucleus for two reasons. First, Hrp38 is predominantly a nuclear protein that binds to the 5′UTR of DE-cadherin presumably in the nucleus. Second, pADPr metabolism is mainly localized in the nucleus. This inference is consistent with a currently accepted model suggesting that IRES transacting factors, such as hnRNPA1, are associated with IRES-containing mRNA in the nucleus from the beginning [38] . However, as recent research has shown that pADPr can regulate microRNA-mediated translation in the cytoplasm [39] , it is entirely plausible that poly(ADP-ribosy)lation also functions in the cytoplasm to inhibit IRES-mediated translation. Our finding that pADPr modification of Hrp38 regulates DE-cadherin expression in the ovary reveals how DE-cadherin expression is regulated during oocyte localization. The localization of the oocyte in the posterior end occurs during the transition from region 2b to region 3 in the germarium [10] . We found that Hrp38 is also expressed in the oocyte and its surrounding follicle cells in region 2b of the germarium ( Fig. 3a ). We also found that the hrp38 mutant has a lower expression of DE-cadherin at the interface between the oocyte and surrounding posterior cells, implying that the hrp38 gene is required for upregulating DE-cadherin expression for oocyte localization. Therefore, we suggest that Hrp38 is required for upregulation of DE-cadherin expression in both the oocyte and surrounding follicle cells by promoting translation ( Fig. 8c ). The expression of Hrp38 in the oocyte and surrounding follicle cells in region 2b helps increase the translation of DE-cadherin by binding to the 5′UTR of DE-cadherin mRNA. The newly produced DE-cadherin assists with anchoring the oocyte in the posterior pole. In mid-body follicle cells and nurse cells, the Hrp38 association with pADPr can downregulate DE-cadherin expression ( Fig. 4e ). As expression of the DE-cadherin transgene in the germline was sufficient to rescue oocyte mislocalization in the Parg mutant double clones ( Fig. 4h ), our finding supports the notion that DE-Cadherin germline mutant clones alone are not sufficient to cause oocyte mislocalization [40] , [41] . In summary, we have identified a pathway that regulates stem cell maintenance and oocyte polarity via pADPr modification of an hnRNP protein (Hrp38) in Drosophila (see Supplementary Discussion for broader implications of these findings). Drosophila strains and genetics Flies were cultured on standard cornmeal–molasses–agar media at 25 °C, unless otherwise indicated. The following stocks were from Bloomington Stock Centre: arm:GAL4/Cyo (#1560); Act5C–GAL4/Cyo (#4414); tubP–GAL4/TM3 (#5538); P{PTT-GC}Hrb98DE ZCL0588 (Hrp38:GFP trap line, #6822); y 1 , w * , v 24 , P{FRT(w hshs ) 101 (#1844). A P-element insertion of the hrp38 gene ( w*,P[XP] d05172 /TM6B, Tb 1 ) and a hrp38 region deficiency line ( w 1118 ; Df(3R)Exel6209, P{XP-U}Exel6209/TM6B, Tb 1 ) from the Exelixis Collection at the Harvard Medical School were replaced with the GFP-bearing balancer ( TM3, P{ActGFP}JMR2, Ser 1 ) for selecting homozygous mutants. Two Hrp38 RNAi lines ( w 1118 ; P{GD14939}v29523 and w 1118 ; P{GD14939}v29524/CyO ) were from the Vienna Drosophila RNAi Centre. The Parg mutant ( Parg 27.1 / FM7, Actin-GFP ) was described previously [42] . The germline-specific GAL4 driver ( nos - Gal4 :VP16) was from Dr Spradling's lab. The BAM-GFP reporter line was a gift from Dr McKearin [27] . The full-length Hrp38 PCR fragment amplified from a hrp38 cDNA clone (LD383464) was cloned into pUAST-RFP (carboxy-terminus fusion) and pUASp-RFP (C-terminus fusion) vectors through the Drosophila Gateway Vector Cloning System (Carnegie Institution of Washington). The full-length DE-cadherin coding region without its 5′UTR was amplified from DE-cadherin cDNA clone (RE37915; DGRC) and cloned into pUASp vector (DGRC). The pUSAp-PARG:EGFP transgene was constructed by cloning the fused fragment of PARG cDNA with EGFP into pUASp vector. All transgenic flies were obtained with the standard P-element-mediated transformation method. Clonal analysis using the FRT-FLP system The Parg female heterozygotes ( Parg 27.1 /FM7a,w a ) were crossed with y 1 , w * , v 24 , P{FRT(w hshs ) 101 /Y [43] to generate the FRT-bearing Parg mutation ( Parg 27.1 , P{FRT(w hshs ) 101 /FM7a,w a ) by genetic recombination. To induce the follicle cell clones in the ovary, Parg 27.1 , P{FRT(w hshs ) 101 /FM7a,w a was crossed with w * , Ubi-GFP, P{FRT(w hshs ) 101 /Y; P{en2.4-GAL4}e16E , P{UAS-FLP1.D}JD1 /Cyo [44] . To induce the Parg mutant germline clones in the ovary, the newly enclosed adults ( Parg 27.1 , P{FRT(w hshs ) 101 /w * , Ubi-GFP, P{FRT(w hshs ) 101 ; P{hs::FLP}38/+) from the progeny of Parg 27.1 , P{FRT(w hshs ) 101 /FM7a crossed with w * , Ubi-GFP,P{FRT(w hshs ) 101 /Y; P{hsFLP}38 (a gift from Dr O'Reilly) were treated by heat-shock at 37 °C for 2 h during the daytime for 2 days. The Parg GSC clones were identified based on the absence of GFP expression and the presence of the round fusome labelled by anti-hts antibody. The wild-type clones were generated using the line ( y 1 , w * , v 24 , P{FRT(w hshs )101) using the same method. The loss rates of the mutant GSCs were counted at 3, 10 and 17 days after clone induction, respectively, based on the published procedure [6] . Biotinylated NAD assay to detect PARP1 activity To detect PARP1 activity in vivo , we used an assay based on incorporation of biotin label donated from b NAD to pADPr proteins [21] , [45] . Biotin incorporation detected after exposure to b NAD is greatly enhanced over intrinsic cytosolic biotin signal. In Drosophila , the utilization of NAD is, in general, PARP1-dependent [21] . To deliver b NAD to tissues for the assay, we dissected Drosophila ovary, leaving exposed tissues in the presence of 2.5 nM b NAD for 1 h. Our previous experiments [21] demonstrate that a period of 30–60 min is sufficient for the detection of PARP1-dependent b NAD utilization. After fixation with 4% paraformaldehyde, we detected the biotin label using Avidin-Rhodamine (Sigma), and visualized biotinylated pADPr by confocal microscopy. Immunohistochemistry Ovaries dissected in Grace's insect medium were fixed in 4% paraformaldehyde+0.1% Triton X-100 in PBS for 20 min and blocked with 0.1% Triton X-100+1% BSA for 2 h. These ovaries were then incubated with the primary antibody overnight at 4 °C, washed three times with PBS+0.1% Triton X-100, and incubated with fluorescence-labelled secondary antibody for 2 h at room temperature. After washing three times with PBS+0.1% Triton X-100, the filamentous actin in the cell membrane was stained with Alexa Fluor 568/633 phalloidin (1:40; Invitrogen) for 30 min, and/or the DNA nuclei were stained with DRAQ5 dye (1:500; Biostatus) for 10 min. The following primary antibodies were used: mouse anti-Orb (4H8, 1:20; DSHB), mouse anti-FasIII (7G10, 1:10; DSHB), mouse anti-Gurken (1D12, 1:10; DSHB), rat anti-DE-cadherin (DCAD2, 1:5; DSHB), rabbit anti-Vasa (1:200; Santa Cruz Biotechnology), mouse anti-hts (1B1,1:20; DSHB), mouse anti-Lamin C (LC28.26, 1:50; DSHB); mouse anti-BAM (1:10; DSHB); rabbit anti-RFP (1:1,000, Clontech). Alexa Fluor 488/568 goat anti-mouse IgG1/Ig2a (1:400; Invitrogen) was used to detect anti-Orb (4H8, IgG1) and anti-FasIII (IgG2a) primary antibodies for double immunostaining. Alexa Fluor 488 goat anti-mouse, Alexa Fluor 568 anti-rabbit and Alexa Fluor 633 anti-rat IgG(H+L) were used to detect other primary antibodies (1:400; Invitrogen). MetaMorph image analysis software (Molecular Devices) was used to quantify the confocal images when required. RNA–protein ultraviolet-crosslinking analysis Biotin-labelled RNA probes were made using 0.2 μg PCR templates amplified from DE-cadherin cDNA clone (RE37915; DGRC) with DIG RNA labelling Kit (Roche). A ultraviolet-crosslinking assay was performed following published methods [46] , [47] with modifications for biotin-labelled probes. The protein lysate from ovaries or the third-instar larvae of the appropriate genotypes was extracted using polysome lysis buffer (100 mM KCl, 5 mM MgCl 2 , 10 mM HEPES, pH 7.0, 0.5% NP-40, 1 mM DTT). The 50 μg lysate was incubated with 40 pg biotin-labelled RNA probe in a 50 μl volume with 5× binding buffer (50 mM Tris-HCl, 250 mM KCl, 5 mM DTT, pH 7.5) on ice for 15 min. The binding reaction was irradiated with 254 nm ultraviolet light for 10 min on ice using Spectrolinker UV Crosslinker (Krackeler Scientific Inc., Albany, NY). The RNA probes were further digested with 10 μg RNAse A (Sigma) and 1,000 U RNAse T1 (Ambion) for 15 min at 37 °C. For IP, the reaction with 150 μl polysome lysis buffer was incubated with the rabbit anti-Hrp38 antibody [34] or rabbit IgG (Sigma; the negative control) at 1:20 dilution overnight and then with 30 μl protein A agarose (Invitrogen) for 2 h at 4 °C. The IP complex was washed using the lysis buffer three times and resolved in 4–12% PAGE gel (Invitrogen). The protein covalently linked to a stub of the biotin-labelled RNA probe was detected with stabilized streptavidin-horseradish peroxidase conjugate with chemiluminescent substrate (Pierce). The blot was stripped and probed with the rabbit anti-Hrp38 antibody (1:10,000). All crosslinking experiments were repeated three times. RNA electrophoretic mobility shift assay RNA electrophoretic mobility shift assay was performed as described earlier [19] . The full-length Hrp38 protein was generated through the cleavage of GST tag by PreScission Protease (GE Healthcare) from GST-Hrp38 recombinant protein, which was expressed from the GST-Hrp38 fusion protein plasmid [34] (a gift from Drs Borah and Steitz). Hrp38 protein was further purified using GSTrap HP columns (GE Healthcare). Either 50 ng GST (BioVision) or 50 ng Hrp38 was incubated with 0.1 μm biotin-labelled G-rich element (413-5′-CAGGGCGCGCACUGUACGAG-3′-432) within the 5′UTR of the DE-cadherin gene (IDT) in binding buffer (Pierce). For the pADPr inhibition assay, 50 ng Hrp38 was preincubated with 140 ng pADPr (Biomol) in 1× binding buffer for 20 min at 25 °C. The experiment was repeated three times. The biotin signals from electrophoretic mobility shift assay were detected with a chemiluminescent kit (Pierce) and measured using the Image J software (NIH). Dual-luciferase reporter assay A bicistronic luciferase reporter plasmid (pMB255) containing Poliovirus IRES element [48] (a gift from Dr Roegiers) was digested with Kpn I and Eco RV to remove Poliovirus IRES completely. DE-cadherin 5′ and 3′UTR PCR products were cloned into the derived luciferase reporter in the forward or reverse orientation. The reporter plasmid (pMB255) was also digested with Eco RV and Pml I and religated as a negative control for firefly luciferase assay. Drosophila S2 cells were maintained at 22 °C in the culture medium supplemented with 10% fetal bovine serum and 1% penicillin/streptomycin. A total of 0.5×10 6 cells per well were seeded into a 6-well plate and incubated for 24 h before the transfection. One microgram of plasmid from the different constructs was transfected into S2 cells using Effectene transfection reagent (Qiagen). After the incubation for 24 h, the firefly and Renilla luciferase activities were measured in triplicate using Dual-Luciferase® reporter assay system (Promega). The ratio of the firefly-to-Renilla luciferase activity was calculated based on experiments performed in triplicate, beginning from the transfection. The statistical analysis was done based on Student's t -test. How to cite this article: Ji, Y. et al . Poly(ADP-ribose) controls DE-cadherin-dependent stem cell maintenance and oocyte localization. Nat. Commun. 3:760 doi: 10.1038/ncomms1759 (2012).